Enantioselective synthesis of tertiary boronic esters through catalytic asymmetric reversed hydroboration Chiral tertiary boronic esters are important precursors to bioactive compounds and versatile synthetic intermediates to molecules containing quaternary stereocenters. The development of conjugate boryl addition to α,β-unsaturated amide has been hampered by the intrinsic low electrophilicity of the amide group. Here we show the catalytic asymmetric synthesis of enantioenriched tertiary boronic esters through hydroboration of β,β-disubstituted α,β-unsaturated amides. The Rh-catalyzed hydroboration occurs with previously unattainable selectivity to provide tertiary boronic esters in high enantioselectivity. This strategy opens a door for the hydroboration of inert Michael acceptors with high stereocontrol and may provide future applications in the synthesis of biologically active molecules. The organoboron compounds have found widespread applications in the design of functional materials and chemical sensors [1] , [2] . In addition, organoborons exhibit important biological properties, including antibacterial, anticancer, and antiviral activities [3] , [4] . These properties have spurred the development of novel therapeutic agents for drug discovery. Moreover, chiral, non-racemic organoboronates are valuable compounds in organic synthesis. A growing list of methods have been developed that enable stereospecific conversion of these compounds to a broad range of functionalized molecules [5] , [6] , [7] , [8] , [9] , [10] , [11] . Tertiary boronic esters are particularly attractive because they provide rapid access to quaternary stereocenters through subsequent transformations [12] , [13] , [14] , [15] , [16] , [17] , [18] , [19] . Pioneering work from Yun [20] , [21] , Shibasaki [22] , [23] , Hoveyda [16] , [24] , [25] , and others [26] , [27] , [28] , [29] , [30] , [31] have established metal-catalyzed boryl conjugate addition as a powerful method for the synthesis of chiral tertiary boronic esters. Starting from α,β-unsaturated compounds, such as ketones and esters, tertiary boronic esters were generated in high enantioselectivities [32] , [33] , [34] . As one of the most important functional groups in organic chemistry, the amide group is ubiquitous in proteins, drugs, and pharmaceutically active compounds [35] , [36] . However, due to the intrinsic low electrophilicity of the amide group, the activity of α,β-unsaturated amide is significantly lower as a Michael acceptor [37] , [38] , [39] . The delocalization of the nitrogen lone pair makes carboxamide the least electron-deficient carboxylic acid derivative. As a result, despite significant advances made in catalytic conjugate additions, currently there are only limited successful examples of catalytic asymmetric conjugate additions to simple α,β-unsaturated amides [40] , [41] , [42] , [43] , [44] , [45] , [46] , and very few of them formed a quaternary stereocenter (Fig. 1a ) [47] . In particular, metal-catalyzed boryl conjugate to simple unsaturated amides has been limited to the synthesis of secondary boronic ester [30] , [48] , [49] , [50] , [51] . There is one example for a copper-catalyzed enantioselective addition to acyclic β,β-disubstituted α,β-unsaturated amide to form a tertiary boronic ester, in which a β-aryl group is necessary to activate the substrate (Fig. 1b ) [52] . Thus, catalytic asymmetric conjugate addition to inert α,β-unsaturated amides to form quaternary stereocenters remains a significant challenge in asymmetric catalysis. A general protocol for catalytic asymmetric hydroboration of β,β-disubstituted α,β-unsaturated amide to form a tertiary boronic ester remains undeveloped. Fig. 1: Catalytic hydroboration of alkenes. a Conjugate addition to α,β-unsaturated amides. b Boryl conjugate addition. c Reversed hydroboration of α,β-unsaturated amides. Full size image We surmised that a metal-catalyzed reversed hydroboration of β,β-disubstituted α,β-unsaturated amide would provide an entry to address this challenge (Fig. 1c ) [53] , [54] , [55] , [56] . In this strategy, a hydride is first incorporated at the α position followed by delivery of the boryl group at the β position, which is mechanistically distinct from a boryl conjugate addition (vide infra). In this type of mechanism, the migratory insertion into the metal hydride by an alkene with low polarity may occur, thus overcoming the inherent low electrophilicity of α,β-unsaturated amide. If the regioselectivity is effectively controlled and the enantioface of the alkene is successfully discriminated, this method would enable facile access to chiral tertiary boronic esters from inert α,β-unsaturated amides. However, we are aware of substantial challenges associated with this design. First, hydroboration of electron-deficient alkenes has been notoriously problematic. Due to the inherent electronic requirement, metal-catalyzed hydroboration of an α,β-unsaturated compound affords a boron enolate [57] , [58] . This type of selectivity has long impeded the development of catalytic enantioselective hydroboration of widely existing electron-deficient alkenes. Second, in addition to the electronic requirement that favors the enolate formation, the steric hindrance at the β position also prefers the addition of a small hydride at this site. The formation of a sterically hindered tertiary boronic ester is disfavored. Third, to obtain high enantioselectivity, the catalyst must be able to differentiate between two similar alkyl groups at the β position in the acyclic system. Therefore, in order to achieve the hydroboration of β,β-disubstituted α,β-unsaturated amide, the catalyst must exert substantial control to override both the electronic and steric preferences, and to obtain high enantioselectivity. We report here a catalytic asymmetric hydroboration of inert α,β-unsaturated amides to construct tertiary boronic esters. The catalyst system we developed is able to (1) reverse the inherent electronic requirement of a hydroboration process, (2) overcome the steric hindrance at the disubstituted β position, and (3) distinguish between the similar steric size of the two β substituents. Starting from easily available materials, this atom-economic process provides a facile method to generate tertiary boronic esters with high regio- and enantioselectivities. This strategy opens a door for the catalytic conjugate addition of inert disubstituted α,β-unsaturated amide to generate quaternary stereocenters. 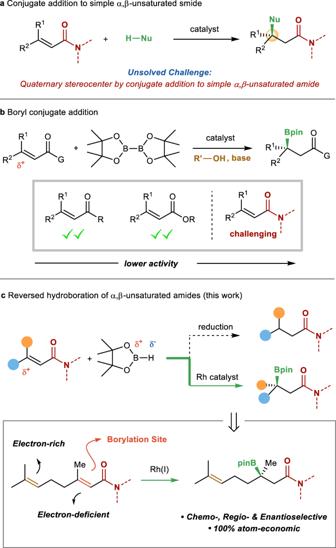Fig. 1: Catalytic hydroboration of alkenes. aConjugate addition to α,β-unsaturated amides.bBoryl conjugate addition.cReversed hydroboration of α,β-unsaturated amides. Reaction development To take advantage of amide as a key designing element [59] , [60] , [61] , [62] , [63] , we began our study by testing the hydroboration of 1a and pinacolborane (HBpin; Table 1 ). In the presence of Rh(COD) 2 OTf, a series of chiral ligands were tested. However, only the reduction product ( 2a ) was detected (entries 1–7). After substantial effort, we found that in the presence of (+)-DIOP ligand L8 (entry 8) [64] , the reversed hydroboration product 3a was obtained in 45% yield together with reduction product. In addition, the tertiary boronic ester was formed in good enantioselectivity. Subsequently, various solvents were tested (entries 9–12). When the reaction was conducted in 1,2-difluorobenzene, the selectivity was improved, favoring the formation of 3a . Lowering the reaction temperature to 0 °C led to an increase ee of 93% (entry 13). Further lowering the temperature to −20 °C increased the enantioselectivity and suppressed the undesired reduction product (entry 14). Interestingly, the addition of catalytic amount of tert -butanol ( t BuOH) further improved the yield (entry 15), although its role in the reaction is still unclear (see the Supplementary information ). Lowering the catalyst loading to 2 mol% did not affect the yield (entry 16). Table 1 Optimization of reaction conditions a . Full size table Reaction scope With this simple yet effective conditions in hand, we investigated the scope of various α,β-unsaturated amides. As summarized in Fig. 2 , α,β-unsaturated amides derived from a variety of amines underwent the reversed hydroboration to give tertiary boronic esters in good yields and high enantioselectivities. The reaction is applicable to substrates derived from both acyclic amines ( 3b – 3d ) and cyclic amines ( 3e – 3k ). The successful hydroboration of Weinreb amide ( 3d ) provides an opportunity to access ketone product. Functional groups, including sulfur, ether, carbamate, and acetal, were compatible with this system ( 3h – 3k ). However, hydroboration of α,β-unsaturated secondary amide with a free NH group did not provide any desired product. Fig. 2: Amide scope. Reversed hydroboration of N -substituted α, β-unsaturated amide. 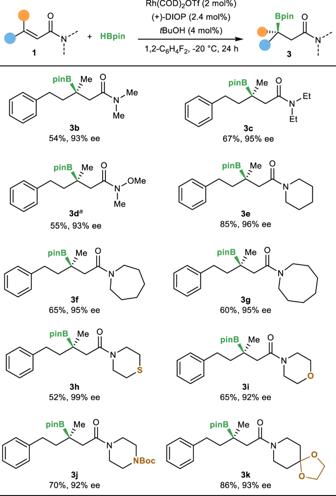Fig. 2: Amide scope. Reversed hydroboration ofN-substituted α, β-unsaturated amide.aThe product was isolated after oxidation. Boct-butyloxy carbonyl. a The product was isolated after oxidation. Boc t -butyloxy carbonyl. Full size image Next, we sought to explore the reversed hydroborations of various β-disubstituted α,β-unsaturated amides (Fig. 3 ). A series of β-disubstituted α,β-unsaturated amides underwent regioselective hydroboration to afford the corresponding products in good yields and high enantioselectivities. Aryl and alkyl halide, ether, silyl ether, ester, and heteroarenes were well compatible with the catalytic system ( 3l – 3y ). The absolute configurations of compounds 3n and 3o were unambiguously confirmed by X-ray crystallography. In addition, the reaction is highly chemoselective, as demonstrated by the preferential reaction of electron-deficient alkene in the presence of electron-rich ones ( 3z , 3aa ). Furthermore, the catalyst system tolerated not only β-methyl substituent, but also larger ethyl and propyl groups ( 3ab , 3ac ). Importantly, the high enantioselectivities obtained by 3ad and 3ae highlighted the ability of the catalyst to differentiate quite similar groups. However, the attempts to form vicinal quaternary and tertiary stereocenters failed despite significant efforts, likely because of the increased steric hindrance ( 3af , 3ag ). Fig. 3: Substrate scope. Reversed hydroboration of β,β-disubstituted α,β-unsaturated amide. a 5 mol% Rh catalyst. b 7.5 mol% Rh catalyst, 3.5 equivalent of HBpin, 0 °C. The product was isolated after oxidation. c 5 mol% Rh catalyst. The product was isolated after oxidation. d 5 mol% Rh catalyst, 6.0 mol% (−)-DIOP. The product was isolated after oxidation. TIPS triisopropylsilyl, MOM methoxymethyl, TBDPS t -butyldiphenylsilyl. Full size image The synthetic utility of this reversed hydroboration was further probed by the reactions of amides derived from drug molecules. Hydroboration of α,β-unsaturated amides derived from tomoxetine, paroxetine, and duloxetine generated the products with high diastereoselectivities ( 3ah , 3ai , 3aj ), no racemization occurred for the existing stereocenters. 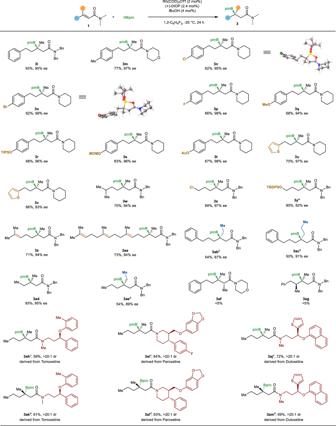Fig. 3: Substrate scope. Reversed hydroboration of β,β-disubstituted α,β-unsaturated amide.a5 mol% Rh catalyst.b7.5 mol% Rh catalyst, 3.5 equivalent of HBpin, 0 °C. The product was isolated after oxidation.c5 mol% Rh catalyst. The product was isolated after oxidation.d5 mol% Rh catalyst, 6.0 mol% (−)-DIOP. The product was isolated after oxidation. TIPS triisopropylsilyl, MOM methoxymethyl, TBDPSt-butyldiphenylsilyl. In addition, the stereoisomers of 3ah , 3ai , 3aj were also obtained with high diastereoselectivities, respectively, when we use (−)-DIOP as the ligand. Transformation of products The resulting reversed hydroboration products could be further transformed to a series of functional groups (Fig. 4 ). For example, enantioenriched tertiary alcohol 4 could be obtained by stereospecific oxidation of the boron compound 3i . Treatment of 3i with KHF 2 yields the potassium trifluoroborate salt 5 in 83% yield. In addition, tertiary boronic esters underwent C–C bond formation with vinyl Grignard or aryl lithium reagent to afford vinylation and arylation compounds 6 and 7 bearing an all-carbon quaternary stereocenter in high enantioselectivities, respectively. Finally, a homologation of the tertiary boronic ester occurred without erosion of the enantioselectivity ( 8 ). Fig. 4: Synthetic utility. Further transformations of the hydroboration products. Reaction conditions: a NaBO 3 , H 2 O, THF; b KHF 2 , MeCN, H 2 O; c (1) vinylMgBr, THF, r.t; (2) I 2 , MeOH, −78 °C; (3) NaOMe, MeOH; d (1) 1-bromo-3,5-dimethoxybenzene, t BuLi, THF, −78 °C; (2) NBS, THF, −78 °C; e (1) ClCH 2 I, n BuLi, THF, −78 °C; (2) H 2 O 2 , NaOH, MeOH, H 2 O. Full size image Mechanistic studies To gain insight into the reaction mechanism, a series of control experiments were performed. First, when α,β-unsaturated ester 9 was used, no reversed hydroboration product 9a was observed under the standard reaction conditions (Fig. 5a ). Thus, the coordinating ability of an amide group plays a crucial role in reaction system. To probe the possibility of a reaction sequence involving alkene isomerization followed by directed alkene hydroboration, catalytic hydroboration of β,γ-unsaturated amides 10 and 11 were conducted. No hydroboration product was observed when using β,γ-unsaturated amide 10 (Fig. 5b ). In addition, the hydroboration of β,γ-unsaturated amide 11 occurred preferentially at the γ position (Fig. 5c ). The β-boration product 3i was obtained in low yield and, more importantly, opposite sense of enantioselectivity. These results provide evidence that the reverse hydroboration occurs directly with α,β-unsaturated amides without prior isomerization. Fig. 5: Control experiments. a Hydroboration of unsaturated ester 9 . b Hydroboration of unsaturated amide 10 . c Hydroboration of unsaturated amide 11 . Full size image Computational studies Computational studies provided information of the energy of each step in the catalytic cycle (Fig. 6 ). Oxidative addition of HBpin to the amide bound rhodium complex ( Int-1 ) generates a five-coordinated rhodium hydride ( Int-2 ). After migratory insertion of the alkene into the rhodium hydride, an alkyl rhodium complex ( Int-3 ) is formed, in which the amide is coordinated to the metal center. Finally, C–B forming reductive elimination delivers the hydroboration product and regenerates the catalyst through ligand exchange. The calculated energies suggest that the migratory insertion is irreversible and determines the enantioselectivity. 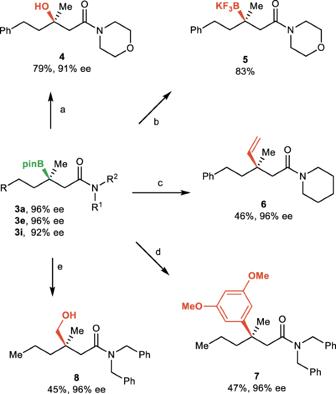Fig. 4: Synthetic utility. Further transformations of the hydroboration products. Reaction conditions:aNaBO3, H2O, THF;bKHF2, MeCN, H2O;c(1) vinylMgBr, THF, r.t; (2) I2, MeOH, −78 °C; (3) NaOMe, MeOH;d(1) 1-bromo-3,5-dimethoxybenzene,tBuLi, THF, −78 °C; (2) NBS, THF, −78 °C;e(1) ClCH2I,nBuLi, THF, −78 °C; (2) H2O2, NaOH, MeOH, H2O. Fig. 6: Proposed mechanism. 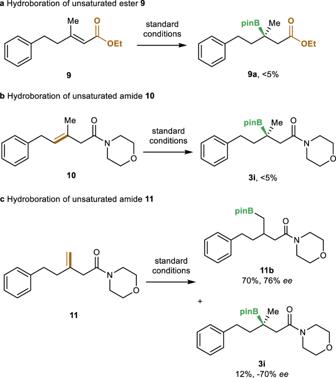Fig. 5: Control experiments. aHydroboration of unsaturated ester9.bHydroboration of unsaturated amide10.cHydroboration of unsaturated amide11. Catalytic cycle with computed free energies of transition states (red) and intermediates (blue) in kcal/mol. Full size image To further understand the origin of enantioselectivity, the energies of different transition states for migration insertion were computed (Fig. 7 ). The lowest energy pathway leading to the S enantiomer has an activation barrier of 21.0 kcal/mol ( TS-2 ), while the lowest energy pathway leading to the R enantiomer has an activation barrier of 23.4 kcal/mol ( TS-2′ ). The energy difference between TS-2 and TS-2′ (2.4 kcal/mol) correlates with the major enantiomer observed in experiments. In TS-2′ , the α,β-unsaturated amide coordinates to rhodium through the opposite enantioface to that in TS-2 . In TS-2 , the phenyl group on the phosphine atom of the ligand forms two attractive CH … O interaction with the carbonyl group of the substrate (CH … O distance 2.26 and 2.45 Å, respectively) [65] , [66] . In contrast, such interaction is not observed in TS-2′ due to the orientation of the carbonyl group. In addition, the phenyl group on the ligand compels the substrate in a way that the ethyl group experiences significant repulsion with the N -methyl group ( TS-2′ ). Therefore, the CH … O interaction with the phenyl group on the ligand in TS-2 and the repulsive interaction in TS-2′ contributes to the relative energies of these transition states, and leads to the high enantioselectivity observed. Fig. 7: Structures of competing transition states. Transition state structures leading to major enantiomer ( TS-2 ) and minor enantiomer ( TS-2′ ). Full size image In summary, we have developed a Rh-catalyzed asymmetric reversed hydroboration to construct chiral tertiary boronic esters. 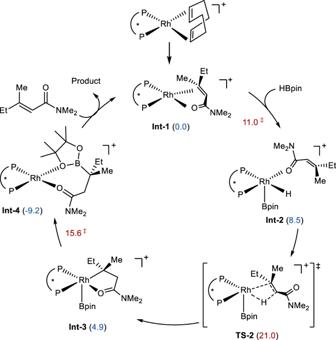Fig. 6: Proposed mechanism. Catalytic cycle with computed free energies of transition states (red) and intermediates (blue) in kcal/mol. 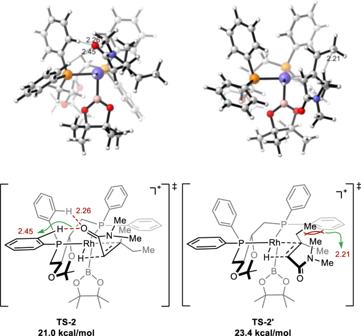Fig. 7: Structures of competing transition states. Transition state structures leading to major enantiomer (TS-2) and minor enantiomer (TS-2′). Using a catalyst formed from cationic rhodium and DIOP ligand, hydroboration of β,β-disubstituted α,β-unsaturated amides delivers chiral tertiary boronic esters with high regioselectivity and enantioselectivity. Computation studies revealed the origin of enantioselectivity. Further mechanistic studies and application of this methodology is ongoing in our laboratory. General procedure for the catalytic hydroboration In an Ar-filled glovebox, the α,β-unsaturated amide (0.25 mmol, 1.0 equiv. ), Rh(COD) 2 OTf (2.3 mg, 2.0 mol%), and (+)-DIOP (3.0 mg, 2.4 mol%) were weighed into a one-dram screw-capped vial. Subsequently, 1,2-difluorobenzene (2.5 mL), t BuOH (4.0 mol%), and pinacolborane (80.0 mg, 2.5 equiv.) were added via syringes. The vial was capped with a Teflon-lined screw cap, and the reaction was then removed from the glovebox and stirred at −20 °C for 24 h. Then the solution was concentrated under reduced pressure. After removal of the solvent, the crude product was analyzed by 1 H NMR and purified by column chromatography on silica gel with EtOAc/hexanes mixture as eluent. Reporting summary Further information on research design is available in the Nature Research Reporting Summary linked to this article.